PRMT9 is a Type II methyltransferase that methylates the splicing factor SAP145 The human genome encodes a family of nine protein arginine methyltransferases (PRMT1–9), whose members can catalyse three distinct types of methylation on arginine residues. Here we identify two spliceosome-associated proteins—SAP145 and SAP49—as PRMT9-binding partners, linking PRMT9 to U2 snRNP maturation. We show that SAP145 is methylated by PRMT9 at arginine 508, which takes the form of monomethylated arginine (MMA) and symmetrically dimethylated arginine (SDMA). PRMT9 thus joins PRMT5 as the only mammalian enzymes capable of depositing the SDMA mark. Methylation of SAP145 on Arg 508 generates a binding site for the Tudor domain of the Survival of Motor Neuron (SMN) protein, and RNA-seq analysis reveals gross splicing changes when PRMT9 levels are attenuated. These results identify PRMT9 as a nonhistone methyltransferase that primes the U2 snRNP for interaction with SMN. Protein arginine methylation is an abundant post-translational modification, with ~0.5% of all arginine residues present in the methylated state in mouse embryonic fibroblasts [1] . Arginine methylation is enriched on RNA-binding proteins [2] , [3] . Indeed, over 50% of the arginine methylation found in mammalian cells is concentrated on heterogeneous nuclear ribonucleoproteins [4] . In addition, a number of well-characterized methylation sites are found on histone tails [5] and splicing factors [6] . Three distinct types of methylated arginine residues occur in mammalian cells. The most prevalent is omega- N G , N G -dimethylarginine [7] . In this case, two methyl groups are placed on one of the terminal nitrogen atoms of the guanidino group; this derivative is commonly referred to as asymmetric dimethylarginine (ADMA). Two other methyl-arginine derivatives occur, namely the symmetrically dimethylated arginine (SDMA) derivative, where one methyl group is placed on each of the terminal guanidino nitrogens, and the omega-monomethylated derivative (ω-MMA). These three types of arginine methylation are catalysed by the nine members of the family of protein arginine methyltransferases (PRMTs) [8] . The PRMTs are classified according to their methylation products [9] . Types I, II and III are able to generate MMA. Type I enzymes include PRMT1, PRMT2, PRMT3, PRMT4/CARM1, PRMT6 and PRMT8, and they all perform a second methylation step to generate the ADMA mark. PRMT5 is the lone Type II enzyme described to date, generating the SDMA mark. PRMT7 is a Type III enzyme and only generates a MMA mark [10] . PRMT9 has not yet been characterized, and it is the subject of this study. PRMT9 has two distinguishing features: (1) similar to PRMT7, it contains an ancestral amino-acid sequence duplication that harbours a second putative S -adenosylmethionine (AdoMet)-binding motif, and (2) unique among the PRMTs, it has three N-terminal tetratricopeptide repeats (TPRs). PRMT9 was identified as a potential human PRMT at the same time as we described PRMT8 (ref. 11 ). In that study, we noted the presence of a gene on chromosome 4q31 encoding a protein most similar to PRMT7 that was relatively well expressed in different tissues and designated it as PRMT9 (ref. 11 ). In the past, the PRMT9 designation has also been used for the product of the human FBXO11 gene on chromosome 2p16 (ref. 12 ), although FBXO11 is unlikely to be a bona fide PRMT [13] . In some literature and protein databases, the gene on human chromosome 4q31 has previously also been referred to as PRMT10, although PRMT9 is the approved symbol and recommended gene name by the HUGO Gene Nomenclature Committee. The characterization of the PRMT9 protein (Q6P2P2 in the UniProt database) has been elusive, mainly because well-known PRMT substrates such as histones and glycine-arginine-rich (GAR) motif-containing proteins are not recognized (or poorly recognized) by the enzyme. Fortuitously, we found that PRMT9 can monomethylate and symmetrically dimethylate a protein that it interacts with, the spliceosome-associated protein, SAP145 (SF3B2). Thus, PRMT9 joins PRMT5 as the only mammalian Type II enzymes. SAP145 is a component of the U2 snRNP (small nuclear ribonucleoprotein) that is recruited to the branch region located near the 3′ splice site, and plays a critical role in the early stages of splicing. We were able to functionally link PRMT9 levels to the regulation of alternative splicing. Thus, we identified PRMT9 as a modulator of the SAP145/SAP49 protein complex that likely plays an important role in snRNP maturation in the cytoplasm. PRMT9 identification and primary sequence features The gene encoding PRMT9 was identified a number of years ago [11] . A scan of the PRMT9 amino-acid sequence for protein domains identified three TPRs at its N terminus ( Supplementary Fig. 1 ). TPRs are helical features that often mediate protein–protein interactions [14] . In addition, similar to PRMT7, PRMT9 harbours two putative AdoMet-binding domains with a clear duplication and partial conservation of most of the six signature PRMT motifs present ( Fig. 1a ). A phylogenetic tree analysis of the encoded amino-acid sequences of all nine members of the PRMT family reveals that it is most closely related to PRMT7 ( Fig. 1b ). The PRMT9 protein, with its defining TPR motifs and ancestrally duplicated sequence, is highly conserved among vertebrates, and is occasionally present in invertebrate animals, but has no orthologues in fungal species or prokaryotes ( Supplementary Fig. 1 ). 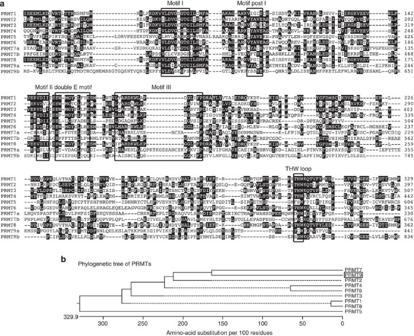Figure 1: Amino-acid sequence alignment of human PRMTs. (a) The amino-acid sequences from the catalytic domain of PRMTs are compared using ClustalW. The signature sequence motifs are boxed with black squares, including the motifs common to seven beta strand enzymes (Motif I, Motif Post I, Motif II and Motif III) as well as the Double E Motif and THW Loop motifs that are specific to PRMTs. The number on the right indicates the positions of amino acid of individual PRMT, starting at the initiator methionine. Human PRMT sequences used included PRMT1: NP_001527.3; PRMT2: NP_996845.1; PRMT3: NP_005779.1; PRMT4: NP_954592.1; PRMT5: NP_006100.2; PRMT6: NP_060607.2; PRMT7: NP_061896.1; PRMT8: NP_062828.3; and PRMT9: NP_612373.2. (b) A straight branched phylogenetic tree of all human PRMTs (shown in phenogram) was generated using ClustalW to demonstrate the evolutionary relationships among these enzymes. Protein sequence accession numbers used in the analysis are listed above. Figure 1: Amino-acid sequence alignment of human PRMTs. ( a ) The amino-acid sequences from the catalytic domain of PRMTs are compared using ClustalW. The signature sequence motifs are boxed with black squares, including the motifs common to seven beta strand enzymes (Motif I, Motif Post I, Motif II and Motif III) as well as the Double E Motif and THW Loop motifs that are specific to PRMTs. The number on the right indicates the positions of amino acid of individual PRMT, starting at the initiator methionine. Human PRMT sequences used included PRMT1: NP_001527.3; PRMT2: NP_996845.1; PRMT3: NP_005779.1; PRMT4: NP_954592.1; PRMT5: NP_006100.2; PRMT6: NP_060607.2; PRMT7: NP_061896.1; PRMT8: NP_062828.3; and PRMT9: NP_612373.2. ( b ) A straight branched phylogenetic tree of all human PRMTs (shown in phenogram) was generated using ClustalW to demonstrate the evolutionary relationships among these enzymes. Protein sequence accession numbers used in the analysis are listed above. Full size image PRMT9 associates with the SAP145 and SAP49 splicing factors To help establish what biological processes PRMT9 may be associated with, we identified proteins that co-purified with PRMT9 expressed in HeLa cells. We performed tandem affinity purification of a TAP-tagged PRMT9 fusion, followed by tryptic digestion and mass spectrometry of the major interacting bands to identify the primary PRMT9 protein complex. The two major interacting proteins were identified as SAP145 and SAP49 ( Fig. 2a ). These splicing factors, also known, respectively, as SF3B2 and SF3B4, are tightly associated with each other [15] . We next developed a monoclonal antibody that specifically recognized the human PRMT9 protein ( Supplementary Fig. 2a–f ). Subcellular localization studies, using this antibody, revealed that PRMT9 is mainly a cytoplasmic protein ( Supplementary Fig. 2d,e ). Using this αPRMT9 antibody and antibodies against endogenous SAP145, we found that PRMT9 and SAP145 were reciprocally co-immunoprecipitated from HeLa cells ( Fig. 2b ). Similarly, green fluorescent protein (GFP)-tagged SAP49 co-immunoprecipitated with endogenous PRMT9 (immunoprecipitating antibodies to endogenous SAP49 are unavailable; Fig. 2c ). To determine whether the interaction between PRMT9 and SAP145 is specific for this arginine methyltransferase, we transfected the complete set of GFP-tagged PRMTs into HeLa cells and immunoprecipitated them. Only GFP-PRMT9 was able to co-immunoprecipitate SAP145 ( Fig. 2d ). We have previously shown that PRMT3 interacts strongly with its substrate, RPS2 (refs 16 , 17 ), and this interaction serves as a control here. 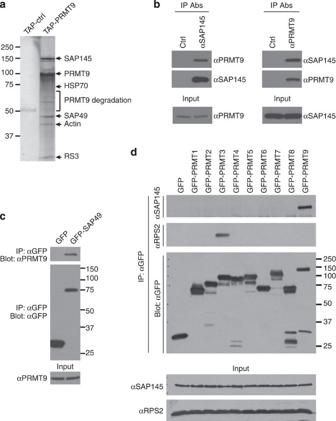Figure 2: PRMT9 interacts with SAP145 and SAP49. (a) TAP-tag purification of the PRMT9 protein complex from HeLa cells. HeLa cells were transiently transfected with either empty TAP-tag vector (TAP-Ctrl) or TAP-tag PRMT9 (TAP-PRMT9). A standard TAP procedure was applied. The eluted protein complex was separated by SDS–PAGE and silver-stained. The indicated gel slices were processed for protein identification using mass spectrometry. Actin, heat-shock protein 70 (HSP70) and 40S Ribosomal Protein S3 (RS3) are likely nonspecific interacting proteins. (b) PRMT9 and SAP145 co-immunoprecipitate. Reciprocal co-IP was performed in HeLa cells. Total cell lysates were immunoprecipitated with rabbit control IgG, αSAP145 antibody (left) and mouse control IgG, αPRMT9 antibody (right). The eluted protein samples were detected by western blotting with αPRMT9 and αSAP145 antibodies. The input samples were detected with αPRMT9 and αSAP145 antibodies, respectively. (c) PRMT9 and SAP49 co-immunoprecipitate. HeLa cells were transiently transfected with either GFP control vector or GFP-SAP49 plasmids. Total cell lysates were immunoprecipitated with αGFP antibody. The eluted protein samples were detected by western blotting with αPRMT9 and αGFP antibodies. The input samples were detected with αPRMT9. (d) Among all the PRMTs, only PRMT9 interacts with SAP145. HeLa cells were transiently transfected with control GFP vector and GFP-PRMTs (1 through 9). The total cell lysates were immunoprecipitated with αGFP antibody. The eluted protein samples were detected by western blotting with αSAP145, αRPS2 and αGFP antibodies. The input samples were detected with αSAP145 and αRPS2 antibodies. Figure 2: PRMT9 interacts with SAP145 and SAP49. ( a ) TAP-tag purification of the PRMT9 protein complex from HeLa cells. HeLa cells were transiently transfected with either empty TAP-tag vector (TAP-Ctrl) or TAP-tag PRMT9 (TAP-PRMT9). A standard TAP procedure was applied. The eluted protein complex was separated by SDS–PAGE and silver-stained. The indicated gel slices were processed for protein identification using mass spectrometry. Actin, heat-shock protein 70 (HSP70) and 40S Ribosomal Protein S3 (RS3) are likely nonspecific interacting proteins. ( b ) PRMT9 and SAP145 co-immunoprecipitate. Reciprocal co-IP was performed in HeLa cells. Total cell lysates were immunoprecipitated with rabbit control IgG, αSAP145 antibody (left) and mouse control IgG, αPRMT9 antibody (right). The eluted protein samples were detected by western blotting with αPRMT9 and αSAP145 antibodies. The input samples were detected with αPRMT9 and αSAP145 antibodies, respectively. ( c ) PRMT9 and SAP49 co-immunoprecipitate. HeLa cells were transiently transfected with either GFP control vector or GFP-SAP49 plasmids. Total cell lysates were immunoprecipitated with αGFP antibody. The eluted protein samples were detected by western blotting with αPRMT9 and αGFP antibodies. The input samples were detected with αPRMT9. ( d ) Among all the PRMTs, only PRMT9 interacts with SAP145. HeLa cells were transiently transfected with control GFP vector and GFP-PRMTs (1 through 9). The total cell lysates were immunoprecipitated with αGFP antibody. The eluted protein samples were detected by western blotting with αSAP145, αRPS2 and αGFP antibodies. The input samples were detected with αSAP145 and αRPS2 antibodies. Full size image Interaction of PRMT9 with SAP145 Next, we mapped the region of SAP145 that interacts with PRMT9. To do this, we broke the SAP145 protein into four roughly equal fragments (F1–4) and expressed them as glutathione S -transferase (GST) fusion proteins ( Fig. 3a ), which we then used to perform a GST pull-down assay with HeLa cell lysates. Western blot analysis revealed that cellular PRMT9 interacts with fragment F3 of SAP145, which encodes for amino acids 401–550 ( Fig. 3b ). This fragment has no distinctive structural features that could help explain the specificity of PRMT9 for this region. We also tested whether the recombinant GST-SAP49 can pull down endogenous PRMT9 using the similar experimental strategy. Interestingly, GST-SAP49 does not interact with PRMT9, suggesting that PRMT9 resides in the SAP145/SAP49 complex through an interaction with SAP145 ( Supplementary Fig. 3a ). We then attempted to perform reciprocal mapping of this interaction to establish which region of PRMT9 associates with SAP145. To do this, we generated a series of flag-tagged PRMT9 deletion constructs ( Supplementary Fig. 3b ). We were particularly interested in the possibility that the TPR motifs would interact with SAP145. However, these motifs proved not to be sufficient for SAP145 binding. Indeed, none of the PRMT9 deletion constructs could interact with SAP145 (or SAP49; Supplementary Fig. 3c ), even though the full-length tagged enzyme retained its binding abilities. This suggests that complete structural integrity of PRMT9 is required to maintain the PRMT9/SAP145/SAP49 protein complex. Supporting this idea, we found that the catalytically inactive form of PRMT9 lost its ability to interact with SAP145 ( Fig. 3c,d ). In addition, while SAP145 and SAP49 were associated with wild-type GFP-PRMT9 expressed in HEK293 cells, neither splicing factor was found to be associated with a catalytically inactive GFP-PRMT9 similarly expressed (data not shown). These results suggest that the integrity of the AdoMet-binding domain of PRMT9 is critical for its interaction with SAP145, and that PRMT9 may release SAP145 after substrate methylation, once it takes on its S -adenosylhomocysteine (AdoHcy)-bound form. Thus, to test whether PRMT9 bound to its product inhibitor AdoHcy would also not interact with SAP145, we treated HeLa cells with adenosine-2',3'-dialdehyde, which results in elevated cellular AdoHcy levels [18] . We then performed a co-immunoprecipitation (co-IP) experiment to evaluate the impact of the AdoMet/AdoHcy switch on the PRMT9/SAP145 interaction. Interestingly, adenosine-2',3'-dialdehyde treatment did not affect the PRMT9/SAP145 interaction, indicating that the AdoHcy-bound form of PRMT9 still likely interacts with its substrate ( Supplementary Fig. 3d ). 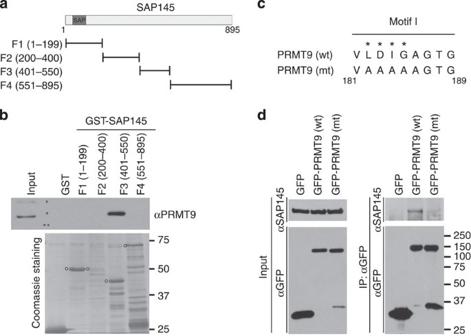Figure 3: Mapping the interaction regions of PRMT9 and SAP145. (a) A series of GST fusion truncations of SAP145 were generated. The location of the SAP (SAF-A/B,Acinus andPIAS) domain is indicated. (b) PRMT9 interacts with the amino acids 401–550 of SAP145. GST pull-down experiment was performed by incubating HeLa cell total lysates with purified GST or GST-tag SAP145 fragments described ina. The pull-down samples were eluted and detected by western blotting using the αPRMT9 antibody. The loading of the proteins was visualized by Coomassie staining of the membrane. The open circles indicate the individual GST-tag SAP145 fragments. (c) Generation of enzymatic mutant PRMT9. The asterisked amino acids (LDIG) located within the conserved Motif I of PRMT9 were mutated to AAAA, causing the loss of methyltransferase activity of enzyme. The numbers below indicate the location of the amino acids on the protein. (d) Wild-type, but not the enzymatic mutant, PRMT9 interacts with SAP145. Co-immunoprecipitation was performed in HeLa cells transiently transfected with GFP control vector, GFP-PRMT9 (wt) and GFP-PRMT9 (mt), as described inc. Total cell lysates were immunoprecipitated with the αGFP antibody. The eluted protein samples were detected by western blotting with αSAP145 and αGFP antibodies. The input samples were detected with αSAP145 and αGFP antibodies as well. Figure 3: Mapping the interaction regions of PRMT9 and SAP145. ( a ) A series of GST fusion truncations of SAP145 were generated. The location of the SAP ( S AF-A/B, A cinus and P IAS) domain is indicated. ( b ) PRMT9 interacts with the amino acids 401–550 of SAP145. GST pull-down experiment was performed by incubating HeLa cell total lysates with purified GST or GST-tag SAP145 fragments described in a . The pull-down samples were eluted and detected by western blotting using the αPRMT9 antibody. The loading of the proteins was visualized by Coomassie staining of the membrane. The open circles indicate the individual GST-tag SAP145 fragments. ( c ) Generation of enzymatic mutant PRMT9. The asterisked amino acids (LDIG) located within the conserved Motif I of PRMT9 were mutated to AAAA, causing the loss of methyltransferase activity of enzyme. The numbers below indicate the location of the amino acids on the protein. ( d ) Wild-type, but not the enzymatic mutant, PRMT9 interacts with SAP145. Co-immunoprecipitation was performed in HeLa cells transiently transfected with GFP control vector, GFP-PRMT9 (wt) and GFP-PRMT9 (mt), as described in c . Total cell lysates were immunoprecipitated with the αGFP antibody. The eluted protein samples were detected by western blotting with αSAP145 and αGFP antibodies. The input samples were detected with αSAP145 and αGFP antibodies as well. Full size image PRMT9 is a Type II PRMT that methylates SAP145 Using in vitro methylation assays with insect cell expressed HA (haemagglutinin)-PRMT9 and the four fragments of SAP145 as potential substrates, we found that only the F3 fragment that physically interacted with PRMT9 ( Fig. 3b ) was also a good methyl-acceptor for the enzyme ( Fig. 4a ). The F2 fragment could not be expressed well, and thus cannot be excluded as a possible substrate. No methylation of the F3 fragment was seen in a similarly expressed PRMT9 enzyme that was mutated in the AdoMet-binding site ( Fig. 4a ). We find that PRMT9 has little or no activity on the typical substrates of other PRMTs including core histones or GAR motif-containing proteins (data not shown). To determine the methylated arginine products of PRMT9, the in vitro 3 H-methylated F3 fragment of SAP145 was subjected to amino-acid analysis. Mammalian expressed GFP-tagged PRMT9 was found to catalyse the formation of both MMA and SDMA only in the presence of the SAP145 fragment ( Fig. 4b ). No methylation was observed in control experiments with the PRMT9 fusion protein mutated in the AdoMet-binding site, demonstrating that the observed activity is intrinsic to tagged PRMT9 and not to another enzyme that might be co-purifying with it ( Fig. 4a,b ). To confirm the formation of SDMA, the radioactive peak from the cation-exchange amino-acid analysis column (corresponding to fractions 57–60) was subjected to thin-layer chromatography under conditions that separated MMA, SDMA and ADMA by their hydrophobic properties. We found that all of the radioactivity comigrated with SDMA ( Fig. 4c ), demonstrating that PRMT9 is a bona fide type II PRMT and joins PRMT5 as only the second enzyme of this type in mammals. A time course of in vitro methylation over a period of 20 h showed a steady accumulation of both MMA and the final product, SDMA ( Supplementary Fig. 4a,b ). 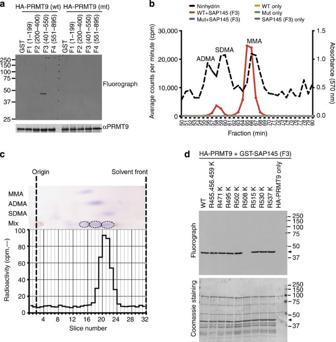Figure 4: PRMT9 catalyses symmetrical dimethylation of SAP145 at Arginine 508. (a) PRMT9 methylates SAP145 fragment F3 (a.a. 401–550). Thein vitromethylation was performed by incubating either wild-type or enzymatic mutant recombinant HA-PRMT9 (purified from Sf21 cells) with GST or GST-tag SAP145 fragments (F1–F4, as described inFig. 3a,b). The loading of PRMT9 was detected by western blotting using the αHA antibody. (b) PRMT9 symmetrically dimethylates SAP145 as detected by amino-acid analysis. Amino-acid analysis ofin vitromethylation products from wild-type and enzymatic mutant GFP-PRMT9 as enzymes and GST-SAP145 (401–550) fragment as substrate. Black dashed line indicates elution of nonradiolabelled standards. The radioactive peaks elute 1–2 min before the nonradiolabelled standards due to a tritium isotope effect39. (c) PRMT9 symmetrically dimethylates SAP145 as detected by thin-layer chromatography (TLC). SDMA fractions from cation-exchange chromatography of thein vitro3H-methylation reaction were separated using TLC. Fractions were spotted on a cellulose plate along with the addition of 5 nmol MMA, 15 nmol ADMA and 5 nmol SDMA internal standards. Individual standards were also spotted in adjacent lanes to determine the migration distance of each methylated arginine derivative. The origin is indicated by fraction 2. The solvent front was run near the end of the plate to fraction 32. The plate was air-dried and each lane was subsequently sliced in 5-mm fractions and counted for three 30-min counting cycles. The radioactive peaks elute 1–2 min before the nonradiolabelled standards due to a tritium isotope effect39. This experiment was repeated three times, and similar migration patterns were observed. (d) PRMT9 methylates SAP145 at R508in vitro. Thein vitromethylation assay was performed by incubating recombinant HA-PRMT9 with a series of Arg to Lys (R to K) mutants of SAP145 fragment F3 (seeFig. 3a,bfor description) for 1 h at 30 °C. After exposure at −80 °C for 3 days, the membrane was stained with Coomassie blue to check the protein loading. Arrows indicate the positions of the substrates and stars indicate the positions of the recombinant HA-PRMT9. Figure 4: PRMT9 catalyses symmetrical dimethylation of SAP145 at Arginine 508. ( a ) PRMT9 methylates SAP145 fragment F3 (a.a. 401–550). The in vitro methylation was performed by incubating either wild-type or enzymatic mutant recombinant HA-PRMT9 (purified from Sf21 cells) with GST or GST-tag SAP145 fragments (F1–F4, as described in Fig. 3a,b ). The loading of PRMT9 was detected by western blotting using the αHA antibody. ( b ) PRMT9 symmetrically dimethylates SAP145 as detected by amino-acid analysis. Amino-acid analysis of in vitro methylation products from wild-type and enzymatic mutant GFP-PRMT9 as enzymes and GST-SAP145 (401–550) fragment as substrate. Black dashed line indicates elution of nonradiolabelled standards. The radioactive peaks elute 1–2 min before the nonradiolabelled standards due to a tritium isotope effect [39] . ( c ) PRMT9 symmetrically dimethylates SAP145 as detected by thin-layer chromatography (TLC). SDMA fractions from cation-exchange chromatography of the in vitro 3 H-methylation reaction were separated using TLC. Fractions were spotted on a cellulose plate along with the addition of 5 nmol MMA, 15 nmol ADMA and 5 nmol SDMA internal standards. Individual standards were also spotted in adjacent lanes to determine the migration distance of each methylated arginine derivative. The origin is indicated by fraction 2. The solvent front was run near the end of the plate to fraction 32. The plate was air-dried and each lane was subsequently sliced in 5-mm fractions and counted for three 30-min counting cycles. The radioactive peaks elute 1–2 min before the nonradiolabelled standards due to a tritium isotope effect [39] . This experiment was repeated three times, and similar migration patterns were observed. ( d ) PRMT9 methylates SAP145 at R508 in vitro . The in vitro methylation assay was performed by incubating recombinant HA-PRMT9 with a series of Arg to Lys (R to K) mutants of SAP145 fragment F3 (see Fig. 3a,b for description) for 1 h at 30 °C. After exposure at −80 °C for 3 days, the membrane was stained with Coomassie blue to check the protein loading. Arrows indicate the positions of the substrates and stars indicate the positions of the recombinant HA-PRMT9. Full size image To localize the site or sites of methylation by PRMT9 on SAP145, each of the 10 arginine residues in the F3 fragment was replaced with a lysine residue. The F3 fragments containing lysine residues at nine of these sites were equally good methyl-acceptors. However, when R508 was mutated to lysine, methylation was greatly diminished, indicating the specificity of PRMT9 for this residue ( Fig. 4d ). Importantly, PRMT9 is an active enzyme when purified from insect cell ( Fig. 4a ) and from mammalian cells ( Supplementary Fig. 5a ), but shows little or no activity when isolated as a GST fusion protein from bacteria ( Supplementary Fig. 5b ). We next tested the ability of a set of eight GST-PRMTs to methylate SAP145-F3. We found that PRMT6 could also readily methylate the F3 fragment, but that no methylation was found with the other enzymes under these conditions ( Supplementary Fig. 5b ). Furthermore, we tested the ability of Myc-PRMT5 (GST-PRMT5 is inactive and was thus not tested in Supplementary Fig. 5b ) to methylate SAP145-F3, and we found that it was unable to do so ( Supplementary Fig. 5C ). Importantly, further analysis using the mutated SAP145-F3 fragments as substrates revealed that PRMT6 mainly methylates the R515 site ( Supplementary Fig. 5d ); therefore, PRMT9 and PRMT6 modify distinct sites on SAP145. Thus, it appears that the SDMA mark at the R508 site of SAP145 is only deposited by PRMT9, and no other Type I or Type II PRMT modifies this site. Reduced PRMT9 levels impact SAP145 methylation To confirm the existence of the SAP145 R508me2s mark in cells, we generated a methyl-specific antibody against this site. Initially, we performed an in vitro characterization of this antibody and we showed that recombinant SAP145-F3 can only be recognized by the αSAP145 R508me2s antibody when it is subjected to prior methylation by PRMT9 ( Fig. 5a ). For immunoreactivity, the methyl-specific antibody also requires the presence of the R508 site. Thus, this antibody is indeed methyl-specific and site-specific ( Fig. 5b ). To establish whether this site is arginine-methylated in cells, we transfected HeLa cells with wild-type or mutant GFP-SAP145 (R508K), and performed western blot analysis with the αSAP145 R508me2s methyl-specific antibody ( Fig. 5c ). The antibody clearly detected the wild-type form of the ectopically expressed fusion protein, but not the mutant form. The endogenous untagged SAP145 protein is also detected as a band that migrates slightly faster than the tagged form. When we repeated this experiment, but co-transfected cells with both SAP145 and PRMT9, we observed a dramatic increase in the levels of the SAP145 methylation as detected with the methyl-specific antibody ( Fig. 5d ). Endogenous SAP145 methylation cannot be further enhanced by PRMT9 overexpression (data not shown), suggesting that endogenous SAP145 is fully methylated at the R508 site. This is not a unique phenomenon for a PRMT substrate, as we have previously shown that poly(A)-binding protein 1 (PABP1) is fully methylated by CARM1, and overexpression of CARM1 cannot further increase the PABP1 methylation level [19] . If this is the case, then the knockdown of PRMT9 should correlate well with the decrease in SAP145 methylation levels, and this is indeed what we observe; endoribonuclease-prepared siRNA (esiRNA)-mediated knockdown of PRMT9 concomitantly reduces the SAP145 methylation level as detected by αSAP145 R508me2s methyl-specific antibody ( Fig. 5e ). 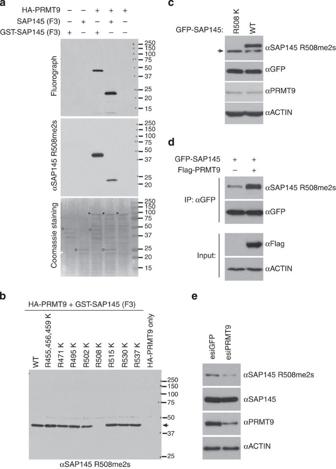Figure 5: PRMT9 symmetrically methylates SAP145 at Arg 508in vivo. (a) SAP145 R508 methylation-specific antibody detectsin vitromethylated SAP145. Thein vitromethylation assay was performed using recombinant HA-PRMT9 as enzyme, either GST-tag SAP145 fragment F3 or SAP145 fragment F3 without GST-tag (cleaved by PreScission Protease) as substrates. The samples were run on a SDS–PAGE gel followed by exposure to X-ray film for 3 days. After exposure, the membrane was stripped and detected using SAP145 R508 methylation-specific antibody (αSAP145 R508me2s) by western blotting. The membrane was then stained with Coomassie blue to check the protein loading. Open circles indicate the positions of the substrates and stars indicate the position of the recombinant HA-PRMT9. (b) Arg to Lys mutation at the R508 site of SAP145 abolishes the recognition of αSAP145 R508me2s antibody. The same membrane, described inFig. 4(d), was stripped and detected using the αSAP145 R508me2s antibody by western blotting. The arrow indicates the position of specific signal detected by the antibody. (c) Arg 508 of SAP145 is symmetrically dimethylated in the cells. HeLa cells were transiently transfected with either GFP-SAP145 or GFP-SAP145 (R508K). 30 μg of total cell lysates were subjected to western blotting detection with αSAP145 R508me2s, αGFP, αPRMT9 and αActin antibodies. The arrow indicates the endogenous SAP145 methylation signals. (d) Overexpression of PRMT9 increases SAP145 R508 symmetrical dimethylation. HeLa cells were transfected with either GFP-SAP145 alone, or GFP-SAP145 and Flag-PRMT9. The total cell lysates were immunoprecipitated with αGFP antibody followed by western blotting with αSAP145 R508me2s and αGFP antibodies. The input samples were detected with αFlag and αActin antibodies. (e) Knockdown of PRMT9 decreases SAP145 R508-symmetric dimethylation. HeLa cells were transiently transfected with either control esiGFP (esiRNA targeting GFP) or esiPRMT9 (esiRNA targeting PRMT9). Total cell lysates (30 μg) were subjected to western blotting and detected with αSAP145 R508me2s, αSAP145, αPRMT9 and αActin antibodies. Figure 5: PRMT9 symmetrically methylates SAP145 at Arg 508 in vivo . ( a ) SAP145 R508 methylation-specific antibody detects in vitro methylated SAP145. The in vitro methylation assay was performed using recombinant HA-PRMT9 as enzyme, either GST-tag SAP145 fragment F3 or SAP145 fragment F3 without GST-tag (cleaved by PreScission Protease) as substrates. The samples were run on a SDS–PAGE gel followed by exposure to X-ray film for 3 days. After exposure, the membrane was stripped and detected using SAP145 R508 methylation-specific antibody (αSAP145 R508me2s) by western blotting. The membrane was then stained with Coomassie blue to check the protein loading. Open circles indicate the positions of the substrates and stars indicate the position of the recombinant HA-PRMT9. ( b ) Arg to Lys mutation at the R508 site of SAP145 abolishes the recognition of αSAP145 R508me2s antibody. The same membrane, described in Fig. 4 ( d ), was stripped and detected using the αSAP145 R508me2s antibody by western blotting. The arrow indicates the position of specific signal detected by the antibody. ( c ) Arg 508 of SAP145 is symmetrically dimethylated in the cells. HeLa cells were transiently transfected with either GFP-SAP145 or GFP-SAP145 (R508K). 30 μg of total cell lysates were subjected to western blotting detection with αSAP145 R508me2s, αGFP, αPRMT9 and αActin antibodies. The arrow indicates the endogenous SAP145 methylation signals. ( d ) Overexpression of PRMT9 increases SAP145 R508 symmetrical dimethylation. HeLa cells were transfected with either GFP-SAP145 alone, or GFP-SAP145 and Flag-PRMT9. The total cell lysates were immunoprecipitated with αGFP antibody followed by western blotting with αSAP145 R508me2s and αGFP antibodies. The input samples were detected with αFlag and αActin antibodies. ( e ) Knockdown of PRMT9 decreases SAP145 R508-symmetric dimethylation. HeLa cells were transiently transfected with either control esiGFP (esiRNA targeting GFP) or esiPRMT9 (esiRNA targeting PRMT9). Total cell lysates (30 μg) were subjected to western blotting and detected with αSAP145 R508me2s, αSAP145, αPRMT9 and αActin antibodies. Full size image The SMN interacts with methylated SAP145 PRMT9 seems to be a rather specific enzyme, and even though many methylated proteins can be detected in HeLa cell extract with pan-MMA and pan-SDMA antibodies, only SAP145 methylation is reduced when PRMT9 levels are lowered ( Supplementary Fig. 6a ). The SAP145 site (R508), which is the target of PRMT9 methylation, is highly conserved in vertebrates and invertebrates ( Supplementary Fig. 6b ), suggesting that it is a critical node of functional control, possibly through the regulation of protein–protein interactions. We first investigated whether methylation of this site regulated the interaction between SAP145 and SAP49. Overexpression of both PRMT9 and SAP145, which causes a dramatic increase in the R508me2s mark ( Fig. 5d ), does not alter the ability of SAP49 to interact with this protein complex ( Supplementary Fig. 6c ). Furthermore, disruption of the R508 methylation site does not affect the assembly of the SAP145/SAP49/PRMT9 complex ( Supplementary Fig. 6d ), suggesting that other protein–protein interactions may be regulated by this mark. Indeed, arginine methylation motifs create docking sites for the recognition by Tudor domain-containing proteins [20] . There are three Tudor domain-containing proteins that are well characterized as effector proteins for methyl-arginine marks, SPF30, Survival of Motor Neuron (SMN) and TDRD3 (ref. 5 ). SMN has been extensively studied and is involved in the assembly of ribonucleoprotein complexes, an important step for snRNP maturation, which regulates mRNA splicing [21] . When we performed a co-IP experiment, we observed the endogenous interaction of SMN with SAP145 ( Fig. 6a ). To address whether the Tudor domain of the SMN protein mediates this interaction, we performed a GST pull-down assay using the Tudor domains from three different proteins (SPF30, SMN and TDRD3). We incubated the GST-tagged recombinant proteins with HeLa cell lysates that were transiently transfected with either wild-type GFP-SAP145 or GFP-SAP145 (R508K) mutant. After pull-down and western blot analysis with αGFP antibody, we observed an interaction between the Tudor domain of SMN and ectopically expressed SAP145, but not with the methylation-deficient SAP145 (R508K; Fig. 6b ). To further confirm this interaction in the cells, we performed co-IP of endogenous SMN with exogenously expressed GFP-SAP145 or GFP-SAP145 (R508K) mutant. Similar to what we observed in the pull-down experiment, endogenous SMN interacts with GFP-SAP145, but not with the methylation-deficient mutant ( Fig. 6c ). To address whether SMN-SAP145 interaction is regulated by PRMT9, we transfected HeLa cells either with GFP-SAP145 alone or with GFP-SAP145 and Flag-PRMT9, followed by a co-IP assay to assess the influence of PRMT9 overexpression on the SMN–SAP145 interaction. Overexpression of PRMT9 dramatically increases the levels of the GFP-SAP145 methylation as detected with the methyl-specific antibody ( Fig. 6d , right panel). Concomitantly, the interaction between SMN and GFP-SAP145 was greatly enhanced ( Fig. 6d , left panel). These results demonstrate that SAP145 R508 methylation by PRMT9 creates a recognition motif for the Tudor domain of SMN, thus facilitating the assembly of the SMN–SAP145 complex. We next investigated whether the SMN–SAP145 interaction is important for U2 snRNP maturation. To do this, we transfected HeLa cells with either GFP-SAP145 or GFP-SAP145 (R508K), and then performed an αGFP immunoprecipitation. An intact methylation site was required for SmB/B′ association with GFP-SAP145, strongly suggesting that the PRMT9 methylation site is critical for SMN-mediated Sm core assembly of the U2 snRNP ( Fig. 6e ). 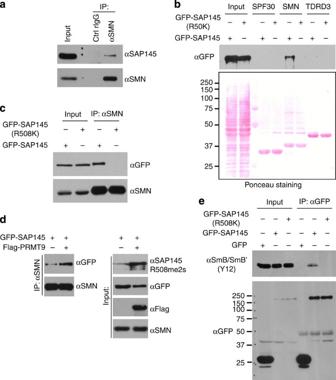Figure 6: Methylation of arginine 508 is required for SAP145–SMN interaction. (a) SMN interacts with SAP145in vivo. Endogenous co-IP was performed by immunoprecipitating HeLa cell nuclear extracts using αSMN antibody, followed by western blotting detection using the αSAP145 antibody. (b) The Tudor domain of SMN interacts with wild-type but not R508K mutant form of SAP145. HeLa cells were transfected with either GFP-SAP145 or GFP-SAP145 (R508K). GST pull-down experiment was performed by incubating transfected cell lysates with recombinant GST-Tudor domains of SPF30, SMN and TDRD3. Eluted samples were detected by western blotting with αGFP antibody. Ponceau S staining displays the loading of total cell lysates and recombinant proteins. (c) SMN interacts with the wild-type but not the R508K mutant form of SAP145. HeLa cells were transfected with either GFP-SAP145 or GFP-SAP145 (R508K). The nuclear extracts were immunoprecipitated with αSMN antibody. The eluted samples and input samples were detected with the indicated antibodies. (d) Overexpression of PRMT9 enhances the interaction of SMN with GFP-SAP145. HeLa cells were transfected with the indicated plasmids. The nuclear extracts were immunoprecipitated with the αSMN antibody. The eluted samples and input samples were detected with the indicated antibodies. (e) An intact SAP145 R508 methylation site is required for U2 snRNP maturation. HeLa cells were transfected with either GFP-SAP145 or GFP-SAP145 (R508K). Cell lysates were immunoprecipitated with the αGFP antibody. The eluted samples and input samples were detected with αSmB (Y12) and with αGFP antibodies. Figure 6: Methylation of arginine 508 is required for SAP145–SMN interaction. ( a ) SMN interacts with SAP145 in vivo . Endogenous co-IP was performed by immunoprecipitating HeLa cell nuclear extracts using αSMN antibody, followed by western blotting detection using the αSAP145 antibody. ( b ) The Tudor domain of SMN interacts with wild-type but not R508K mutant form of SAP145. HeLa cells were transfected with either GFP-SAP145 or GFP-SAP145 (R508K). GST pull-down experiment was performed by incubating transfected cell lysates with recombinant GST-Tudor domains of SPF30, SMN and TDRD3. Eluted samples were detected by western blotting with αGFP antibody. Ponceau S staining displays the loading of total cell lysates and recombinant proteins. ( c ) SMN interacts with the wild-type but not the R508K mutant form of SAP145. HeLa cells were transfected with either GFP-SAP145 or GFP-SAP145 (R508K). The nuclear extracts were immunoprecipitated with αSMN antibody. The eluted samples and input samples were detected with the indicated antibodies. ( d ) Overexpression of PRMT9 enhances the interaction of SMN with GFP-SAP145. HeLa cells were transfected with the indicated plasmids. The nuclear extracts were immunoprecipitated with the αSMN antibody. The eluted samples and input samples were detected with the indicated antibodies. ( e ) An intact SAP145 R508 methylation site is required for U2 snRNP maturation. HeLa cells were transfected with either GFP-SAP145 or GFP-SAP145 (R508K). Cell lysates were immunoprecipitated with the αGFP antibody. The eluted samples and input samples were detected with αSmB (Y12) and with αGFP antibodies. Full size image PRMT9 is required for efficient alternative splicing The robust and specific interaction between PRMT9 and SAP145/SAP49 ( Fig. 2 ), the ability of PRMT9 to methylate SAP145 ( Fig. 4 ) and the regulation of methylation-dependent SMN–SAP145 interaction by PRMT9 ( Fig. 6 ) strongly suggest that PRMT9 is involved in the regulation of mRNA splicing. To investigate this possibility, we extracted total RNA from control knockdown and esiRNA-mediated PRMT9 knockdown HeLa cells and subjected them to RNA-sequencing (RNA-seq) analysis, particularly focusing on changes in alternatively spliced events. To reduce the experimental variation, two sets of biological replicates were prepared. Western blot analysis demonstrated the efficient knockdown of endogenous PRMT9 in both replicate samples ( Fig. 7a ). For RNA-seq, we performed 75-nt paired-end sequencing and achieved ~220 million and 120 million unique mapped reads for control knockdown and PRMT9 knockdown, respectively. We used a mixture-of-isoform (MISO) model 2 to compute and quantify alternative splicing events. We were able to identify five types of alternative splicing events, which were significantly altered. These events included 34 skipped exons, 13 retained introns, 9 alternative 3′ splice sites, 9 alternative 5′ splice sites and 3 mutually exclusive exons ( Supplementary Table 1 ). One example of the MISO output landscape is displayed in Fig. 7b , showing RNA-seq read coverage across EDEM1 exon 8 to exon 10 from esiGFP control and esiPRMT9 knockdown HeLa cells. To validate the alternative splicing called by MISO, reverse transcription–polymerase chain reaction (RT–PCR) was performed using the primers located within the flanking exons of the EDEM1 gene. Knockdown of PRMT9 using esiRNA reduces the inclusion/exclusion ratio to ~2.5-fold ( Fig. 7c ). At another gene loci ( NGLY1 ), knockdown of PRMT9 expression increases the inclusion/exclusion ratio to ~2.5-fold ( Supplementary Fig. 7a,b ). It should be noted that esiRNA-mediated knockdown of PRMT9 only causes an ~50% decrease in the SAP145 R508 methylation level ( Fig. 5e ). A small amount of enzyme is still capable of carrying out substantial methylation. This may explain why we can only capture a small group of altered splicing events. Total removal of PRMT9 may have more profound effects on alternative splicing. Thus, PRMT9 is having an impact on alternative splicing in a number of different ways, possibly through its ability to methylate SAP145 and promote the interaction between SAP145 and SMN. 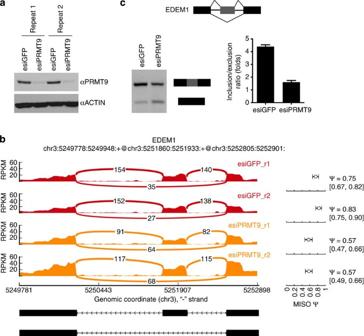Figure 7: PRMT9 regulates alternative splicing. (a) Two sets of biological replicated samples for RNA-seq. HeLa cells were transiently transfected with esiGFP control or esiPRMT9. The total RNA was extracted 72 h after transfection. Western blotting confirms the knockdown of the PRMT9 protein using αPRMT9 and αActin antibodies. (b) RNA-seq read coverage across EDEM1 exon 8 to exon 10 from esiGFP control and esiPRMT9 knockdown HeLa cells. MISO (Ψ) values and 95% confidence intervals were shown at right. (c) Validation of exon exclusion of EDEM1 exon 9 in response to PRMT9 knockdown. RT–PCR experiments were performed using RNA extracted from esiGFP control and esiPRMT9-transfected HeLa cells with primers located on exon 8 and exon 10 (left panel). The PCR products were quantified using the densitometric analysis. Inclusion versus exclusion ratio was calculated. Error bars represent s.d. calculated from three independent experiments (right panel). Figure 7: PRMT9 regulates alternative splicing. ( a ) Two sets of biological replicated samples for RNA-seq. HeLa cells were transiently transfected with esiGFP control or esiPRMT9. The total RNA was extracted 72 h after transfection. Western blotting confirms the knockdown of the PRMT9 protein using αPRMT9 and αActin antibodies. ( b ) RNA-seq read coverage across EDEM1 exon 8 to exon 10 from esiGFP control and esiPRMT9 knockdown HeLa cells. MISO ( Ψ ) values and 95% confidence intervals were shown at right. ( c ) Validation of exon exclusion of EDEM1 exon 9 in response to PRMT9 knockdown. RT–PCR experiments were performed using RNA extracted from esiGFP control and esiPRMT9-transfected HeLa cells with primers located on exon 8 and exon 10 (left panel). The PCR products were quantified using the densitometric analysis. Inclusion versus exclusion ratio was calculated. Error bars represent s.d. calculated from three independent experiments (right panel). Full size image We have demonstrated that PRMT9 is a Type II enzyme using both amino-acid analysis approaches and methyl-specific antibodies that recognize the SDMA mark on SAP145. It is unclear how many additional substrates PRMT9 might have; however, it is likely not as promiscuous as PRMT5, which methylates a broad swath of GAR motif-containing proteins. PRMT5 is the founding member of the Type II class of PRMTs, and clearly the dominant enzyme in this class. When cell lysates are subjected to western blot analysis using pan-SDMA antibodies, the majority of the bands detected in wild-type cells are lost in PRMT5 knockdown cell lines [1] . Quantification of the different types of arginine methylation across a large number of tissue and cell types have estimated the ratios to be roughly 1,500:3:2:1 for Arg:ADMA:MMA:SDMA [1] , [7] , [22] . Measurements of cellular SDMA levels using PRMT5 knockout (KO) cells are yet to be performed; however, this would establish what proportion of the SDMA is deposited by PRMT5 and PRMT9, respectively. Although PRMT5 and PRMT9 are both Type II enzymes, they do not display redundancy. In in vitro methylation assays these two PRMTs do not recognize each other’s substrates ( Supplementary Fig. 5c and data not shown). In addition, subsets of SDMA-specific antibodies selectively recognize PRMT5 or PRMT9 substrates as validated using the respective knockdown cell extracts (data not shown). The extended seven-amino-acid (CFKRKYL) PRMT9 methylation motif in SAP145 ( Supplementary Fig. 6b ) is not found in any other protein. However, when we reduce the search to a five-amino-acid motif (FKRKY) we did identify eight human proteins that could possibly be substrates for this newly characterized enzyme, and they will be tested in the near future. After we designated the gene on human chromosome 4q31 as PRMT9 (ref. 11 ), this designation was also used for the FBXO11 gene on human chromosome 2p16 (ref. 12 ). FBXO11 does not contain the signature amino-acid sequence motifs of the PRMT family and the description of its activity as a PRMT likely was the result of contamination of the FLAG-tagged protein with PRMT5 (ref. 12 ). No methyltransferase activity has been observed with the nematode homologue of FBXO11 (ref. 13 ). It has been clearly shown that the monoclonal M2 antibody used to pull down FLAG-tagged proteins will also bring down endogenous PRMT5, thus contaminating any preparation of a FLAG-tagged protein [9] , [23] . Owing to the usage of PRMT9 for both of these gene products, PRMT10 has also been used to designate the 4q31 product. However, PRMT9 is now the approved symbol and recommended gene name by the HUGO Gene Nomenclature Committee for the PRMT characterized in this work. Classic studies in the arginine methylation field first implicated this post-translational modification in the regulation of RNA metabolism [3] , [4] . More recently, large-scale proteomic analysis of arginine-methylated proteins revealed the identity of many of these RNA-binding proteins [24] , [25] . Both Type I and Type II PRMTs are involved in the regulation of splicing. The Type I enzyme, CARM1, enhances exon skipping in an enzyme-dependent manner [6] , [26] . It regulates splicing by methylating a number of splicing factors (CA150, SAP49, SmB and U1C), likely at transcriptionally active sites to which it is recruited as a transcriptional coactivator [6] . PRMT6 is another transcriptional co-regulator that does not exclusively modulate gene expression, but also has an impact on alternative splicing patterns [27] . Indeed, transcriptome analysis of PRMT6 knockdown cells revealed a number of gene-specific exon pattern changes, including altered exon retention and exon skipping [28] . The Type II enzyme, PRMT5, functions as a transcriptional repressor in the nucleus by symmetrically methylating histone H4R3 and H3R8 (ref. 29 ). In the cytoplasm, PRMT5 is primarily found in the 20S methylosome complex, along with MEP50, pICIn and various Sm proteins (SmB/B′, D1–3, E, F and G) [30] , [31] , [32] . In this complex, the Sm proteins are symmetrically dimethylated by PRMT5. In turn, the methylated Sm proteins interact with the Tudor domain of SMN [33] , which helps to load the Sm proteins on spliceosomal snRNAs (U1, U2, U4, U5, U11 and U12) [21] , [34] . Thus, PRMT5 plays a critical role in spliceosomal U snRNP maturation. PRMT5 has a rather central role in pre-mRNA splicing, and it is assumed that pleiotropic splicing defects will be observed on PRMT5 loss; this is indeed the case. The conditional removal of PRMT5 in mouse neural progenitor cells results in defects in both constitutive splicing and alternative splicing [35] . Furthermore, in Arabidopsis , PRMT5 is essential for proper pre-mRNA splicing [36] , [37] . The splicing factors SAP145 and SAP49 are tightly associated with each other [15] . SAP145 and SAP49 are dedicated components of the nuclear U2 snRNP. The region of SAP145 that interacts with SAP49 has been mapped, and it lies adjacent to the R508me2s site [38] . Methylation of R508 does not have an impact on the SAP145/SAP49 interaction ( Supplementary Fig. 6 ). The PRMT9/SAP145/SAP49 complex likely forms in the cytoplasm, where PRMT9 deposits the SAP145 R508me2s mark for subsequent recognition by SMN. In mammals, newly synthesized snRNAs are first exported to the cytoplasm, where they undergo maturation (partial snRNP complex assembly) before being imported back into the nucleus to form catalytically active snRNPs [21] . As described above, PRMT5 plays a critical role in the biogenesis of the Sm-class of spliceosomal snRNPs. PRMT9 seems to add another level of maturation, which is specific for U2 snRNA. A fairly unique feature of PRMT9 is its ability to strongly interact with its substrate, SAP145 ( Fig. 2d ); most PRMTs, with the exception of PRMT3, do not do this. The PRMT9/SAP145 interaction occurs in the cytoplasm. However, copious quantities of SAP145 are observed in the nucleus [38] . Thus, it is likely that some signals, perhaps a post-translational modification, regulate the dissociation of PRMT9 and SAP145 to facilitate nuclear translocation of the maturing U2 snRNP. Indeed, we observe reduced SmB/B′ association with mutant SAP145 (GFP-SAP145 R508K ), which is indicative of an U2 snRNP maturation defect. This flaw in U2 snRNP maturation could modify the fidelity of branch point recognition and alter a subset of alternative splicing events. Plasmids and antibodies Human PRMT9 cDNA (NM_138364.2) was subcloned into a pGEX-6p-1 vector (GE Healthcare Life Sciences), a pEGFP-C1 vector (Clontech) and a 3XFlag vector (Invitrogen). NTAP-PRMT9 used for tandem affinity purification was generated by cloning human PRMT9 cDNA into pCeMM NTAP(GS) vector (EUROSCARF). Human SAP49 cDNA, SAP145 cDNA and its truncated cDNAs were cloned into pEGFP-C1 vector. Both wild-type and mutant HA-PRMT9 were cloned into pBacPAK vector (Clontech) for insect cell expression. Rabbit anti-GFP polyclonal antibody was purchased from Invitrogen (Cat no. A6455, used for IP, 2 μl per IP). Mouse anti-HA monoclonal antibody was purchased from Covance (Cat no. MMS-101P-200, used for western blot, 1:2,000 dilution). Mouse anti-Flag M2 monoclonal antibody was purchased from Sigma (Cat no. A2220, used for IP, 20 μl per IP). Rabbit anti-SAP145 polyclonal antibody was purchased from Novus Biologicals (Cat no. NB100-79848 used for western blot analysis, 1:3,000 dilution and IP, 5 μl per IP). Rabbit anti-SAP49 polyclonal antibody was purchased from Abcam (Cat no. ab66659, used for western blot analysis, 1:1,000 dilution). Mouse anti-PRMT9 monoclonal antibody was raised, using the recombinant GST-PRMT9 as antigen, by the Antibody Facility Core at M.D. Anderson Cancer Center (used for western blot analysis, 1:1,000 dilution and IP, 10 μl per IP). The SAP145 R508me2s antibody was identified in a screen for SDMA-specific antibodies (used for western blot, 1:1,000 dilution). Cell Signaling Technology generated this panel of antibodies using the XXXXR me2s XXR me2s XXXXR me2s XXXR me2s XXXX peptide as an antigen. The resulting antibodies were screened on PRMT5 KO cells, and the majority displayed a loss of immunoreactivity. However, two of these antibodies, BL8244 and BL8245, strongly recognized a band of roughly 150 kDa, which is not lost in PRMT5 KO cells. When we tested these two antibodies on PRMT9 knockdown cells, the immunoreactivity of this 150-kDa band was reduced. We thus went on to characterize these antibodies in vitro ( Fig. 5 ). Uncropped immunoblots for each figure are shown in Supplementary Fig. 8 . Tandem affinity purification HEK293 cells (from ATCC) were transfected with NTAP-PRMT9. A total of 1 × 10 8 cells were used for tandem affinity purification. In brief, cells were first lysed in lysis buffer containing 50 mM Tris-HCl (pH 7.5), 125 mM NaCl, 5% glycerol, 0.2% NP-40, 1.5 mM MgCl 2 , 25 mM NaF, 1 mM Na 3 VO 4 and protease inhibitors. After centrifugation at maximum speed for 10 min, the supernatant was incubated with rabbit-IgG Sepharose (GE Healthcare Life Sciences) at 4 °C for 4 h. The bound beads were first washed with lysis buffer and then with TEV-protease cleavage buffer (10 mM Tris-HCl (pH 7.5), 100 mM NaCl and 0.2% NP-40). The bound protein complexes were eluted by addition of 50 μg TEV protease (4 °C, overnight). TEV-protease cleavage products were then incubated with Streptavidin agarose (Millipore) at 4 °C for 2 h. The bound proteins were heated at 100 °C for 5 min in SDS sample buffer and analysed using SDS–PAGE followed by either silver staining or SYPRO Ruby staining. After comparison with the control samples, differentially expressed bands were cut from the gel and proteins were identified with liquid chromatography-tandem mass spectrometry (LC-MS/MS) using the Protein and Metabolite Analysis Core Facility at UT Austin. Baculovirus expression and protein purification HA-PRMT9 (both wild-type and the enzymatic mutant as described below) in pBacPAK8 vector were co-transfected with linearized Baculovirus DNA (BD Biosciences) using the FuGENE 6 transfection reagent (Roche). The expression and purification of recombinant proteins were followed according to the instruction manual of Baculovirus Expression Vector System (6th Edition, May 1999), except that HA-conjugated beads and HA peptide (Sigma) were used to bind and elute the recombinant proteins, respectively. Purified proteins were then dialysed in 1 × TBS buffer (50 mM Tris-Cl, pH 7.5, 150 mM NaCl) and used for the in vitro methylation assay. Immunoprecipitation HeLa cells were washed with ice-cold PBS and lysed with 1 ml of co-IP buffer (50 mM Tris-HCl (pH 7.5), 150 mM NaCl, 0.1% NP-40, 5 mM EDTA, 5 mM EGTA, 15 mM MgCl 2 ) with protease inhibitor cocktail. After sonication, insoluble materials were removed by centrifugation at maximum speed for 10 min. Whole-cell lysates were incubated with 2 μg of immunoprecipitation antibody overnight. After incubation with Protein A/G agarose beads, the bound proteins were eluted and analysed using western blot analyses. Immunofluorescence HeLa cells (from ATCC) were grown on glass coverslips to desired confluence before fixation. Cells were rinsed with PBS and fixed with 4% paraformaldehyde for 15 min at room temperature. After blocking with 20% newborn calf serum, cells were incubated with monoclonal PRMT9 antibody (1:1,000) at 4 °C overnight. Cells were then stained with secondary antibody and DAPI sequentially. The coverslips were then sealed and examined under a NIKON Eclipse E800 fluorescent microscope. GST pull down GST and different recombinant proteins were expressed and purified from Escherichia coli . The individual protein was incubated with HeLa cell lysates at 4 °C overnight. The protein complex was then incubated with Glutathione Sepharose 4B resin (GE Healthcare Life Sciences) for 1 h at 4 °C. The eluted samples were loaded on SDS–PAGE gel and detected with western blot analyses using the indicated antibodies. Equal loading of the recombinant proteins was visualized by either Coomassie blue staining or ponceau staining. Nuclear and cytoplasmic extraction Cytoplasmic and nuclear fractions of HeLa cells were extracted following the protocol as described in the instructions from the NE-PER Nuclear and Cytoplasmic Extraction Kit (Pierce Biotech). esiRNA knockdown esiRNA used for transient knockdown of PRMT9 was designed using the website http://cluster-12.mpi-cbg.de/cgi-bin/riddle/search . The preparation of dsRNA was followed according to the instructions of the MEGAscript RNAi Kit (Invitrogen). dsRNA was then digested with RNase III to produce a blender of 18- to 30-bp siRNA mixture. After purification, the esiRNA was dissolved in H 2 O and tested for knockdown efficiency. Site-directed mutagenesis Human PRMT9 was mutated to create a catalytically inactive mutant by introducing quadruple mutations (L182A, D183A, I184A and G185A) in the conserved motif I in both the HA-PRMT9 and GFP-PRMT9 plasmid vectors. Mutant primers (IDT, San Diego, CA) were as follows: forward 5′- TGTTTGGGGTCCAAAAGTGTTGCGGCCGCTGCGGCAGGAACTGGAATACTAAGC -3′ and reverse primer 5′- GCTTAGTATTCCAGTTCCTGCCGCAGCGGCCGCAACACTTTTGGACCCCAAACA -3′ ( T m=86.7 °C). PCR reactions were set up according to the QuikChange XL Site-Directed Mutagenesis kit (Agilent Technologies Inc.). GST-SAP145 Arginine to Lysine series mutants were generated using the same strategy. All mutations were confirmed on positive colonies by DNA sequencing. In vitro methylation assay In vitro methylation reactions were carried out in 30 μl of PBS (pH=7.4.) containing 0.5–1.0 μg of substrate, 3 μg of recombinant enzymes and 0.42 μM S-adenosyl-l-[methyl- 3 H]methionine (79 Ci mmol −1 from a 7.5 μM stock solution; PerkinElmer Life Sciences). The reaction was incubated at 30 °C for 1 h and then separated on SDS–PAGE, transferred to a polyvinylidene difluoride membrane, treated with En3Hance (PerkinElmer Life Sciences) and exposed to a film for 1–3 days at –80 °C. High-resolution cation-exchange chromatography In vitro methylation reactions were set up with ~2 μg of enzyme protein, ~5 μg of substrate and 0.7 μM S -adenosyl-L-[ methyl - 3 H]methionine (PerkinElmer Life Sciences, 75-85 Ci mmol −1 , 0.55 mCi ml −1 in 10 mM H 2 SO 4 /EtOH (9:1, v/v)) in a final reaction volume of 60 μl. The reactions were incubated and rotated for 1, 5 or 20 h at 37 °C, in a reaction buffer of 50 mM potassium HEPES, 10 mM NaCl and 1 mM dithiothreitol, pH 8.0. To quench the reaction, a final concentration of 12.5% trichloroacetic acid was added with 20 μg of the carrier protein bovine serum albumin. After a 30-min incubation at room temperature, the precipitated proteins were centrifuged at 4,000 × g for 30 min and washed with cold acetone to remove excess [ 3 H]AdoMet, and the pellet was air-dried before acid hydrolysis. Fifty microlitres of 6 N HCl were added to each dried pellet, and 200 μl of 6 N HCl was added to a Waters PicoTag Chamber. Each sample was acid-hydrolysed in vacuo at 110 °C for 20 h. After acid hydrolysis, the pellets were dried using vacuum centrifugation. To prepare samples for high-resolution cation-exchange chromatography, the hydrolysed samples were resuspended in 50 μl of water and mixed with sodium citrate buffer (0.2 M in Na+, pH 2.2) and standards including 1 μmol each of ω-MMA (acetate salt, Sigma, M7033), SDMA (di(p-hydroxyazobenzene)-p′-sulfonate salt, Sigma, D0390) and ADMA (hydrochloride salt, Sigma, D4268). Samples were loaded on sulfonated polystyrene resin and eluted using 0.35 M sodium citrate running buffer, pH 5.25, at 55 °C. One-milliliter fractions were collected and the positions of the internal standards were determined using a ninhydrin assay using only 50 μl of each fraction. Fractions (950 μl) were assayed for radioactivity by the addition of 10 ml of Safety Solve Scintillation cocktail (Research Products International, 111177) and data were reported as the average of three 5-min counting cycles on a Beckman LS6500 Liquid Scintillation instrument. Thin-layer chromatography Fraction samples were spotted on a cellulose plate along with the addition of 5 nmol MMA, 15 nmol ADMA and 5 nmol SDMA of internal standards as described above. Individual standards were also spotted in adjacent lanes to determine the migration distance of each methylated arginine derivative. The origin is indicated by fraction 2. The solvent front was run near the end of the plate to fraction 32. The plate was air-dried and each lane was subsequently sliced in 5-mm fractions and counted using liquid scintillation counting for three 30-min counting cycles. This experiment was repeated three times and similar migration patterns were observed. Protein sequence alignment using ClustalW The parameters for the alignment using ClustalW were set as follows: Gap Penalty: 10, Gap Length Penalty: 0.2, Delay Divergent Seqs (%) 30, Protein Weight Matrix: Gonnet Series for multiple alignment parameters, and for pairwise alignment, Gap Penalty: 10, Gap Length 0.1, Protein Weight Matrix: Gonnet 250. Deep-sequencing and alternative splicing analysis by MISO Paired-end strand-specific RNA-seq reads were aligned to the human genome (hg19) using TopHat 2.0.91. We performed 75-nt paired-end sequencing and achieved ~220 million and 120 million unique mapped reads for control knockdown and PRMT9 knockdown, respectively. On the basis of the alignment result from TopHat, MISO model2 was used to compute ‘percentage spliced in’ (PSI or Ψ ) values to quantify alternative splicing, indicating the fraction of a gene’s mRNAs that include the alternative region. Five types of alternative splicing were analysed, including skipped exons, alternative 3′/5′ splice sites, mutually exclusive exons and retained intron. Then, change of Ψ and Bayes factor (>10) was used to identify significantly altered splicing in PRMT9 knockdown. Accession codes: Deep-sequencing data can be accessed with GEO accession number GSE63953 . How to cite this article: Yang, Y. et al . PRMT9 is a Type II methyltransferase that methylates the splicing factor SAP145. Nat. Commun. 6:6428 doi: 10.1038/ncomms7428 (2015).